The MST1/2-SAV1 complex of the Hippo pathway promotes ciliogenesis Primary cilia are microtubule-based organelles that protrude from polarized epithelial cells. Although many structural and trafficking molecules that regulate ciliogenesis have been discovered, signalling proteins are not well defined. Here we show that the MST1/2-SAV1 complex, a core component of the Hippo pathway, promotes ciliogenesis. MST1 is activated during ciliogenesis and localizes to the basal body of cilia. Depletion of MST1/2 or SAV1 impairs ciliogenesis in cultured cells and induces ciliopathy phenotypes in zebrafish. MST1/2-SAV1 regulates ciliogenesis through two independent mechanisms: MST1/2 binds and phosphorylates Aurora kinase A (AURKA), leading to dissociation of the AURKA/HDAC6 cilia-disassembly complex; and MST1/2-SAV1 associates with the NPHP transition-zone complex, promoting ciliary localization of multiple ciliary cargoes. Our results suggest that components of the Hippo pathway contribute to establish a polarized cell structure in addition to regulating proliferation. Primary cilia are microtubule-based organelles that extrude from the apical surface of epithelial cells and function as antennae that monitor the extracellular environment [1] . Primary cilia recognize physical cues, such as flow of extracellular fluid, and interpret them to regulate cell growth and proliferation [2] . They also receive various chemical cues, such as Shh, Notch or PDGFA, by concentrating the cognate receptors and signalling proteins within the cilia [3] , [4] . Given the diverse roles of cilia, humans with defective ciliogenesis develop multiple diseases (ciliopathies) with a broad range of pathological symptoms [5] . These observations underscore the importance of understanding how ciliogenesis is regulated. As the basal body and the centrosome share the centriole as a microtubule-organizing centre, ciliogenesis is tightly coupled with the cell cycle [6] . Upon cell-cycle exit, the centriole moves to the apical membrane, docks beneath it and transforms into the basal body through a complex re-organization of associated proteins. When cells encounter cell-cycle re-entry cues, the cilia disassemble and the basal body transforms back to a centrosome to provide the mitotic spindles required for the next mitosis. Most of the factors implicated in ciliogenesis are scaffold proteins, structural components of the cilia or trafficking proteins. However, the signalling proteins involved in ciliogenesis, such as kinases, phosphatases and ubiquitination system proteins, are less defined. It has been suggested that the AURKA/HDAC6 pathway mediates cilia disassembly [7] . Upon receiving a cell-cycle re-entry cue, Aurora kinase A (AURKA) is activated and in turn enhances the activity of HDAC6, an enzyme that deacetylates ciliary tubulin, promoting cilia disassembly. Several mechanisms have been proposed for regulation of AURKA activity during cilia disassembly, including stabilization of AURKA itself; interaction with activating scaffold proteins, such as NEDD9 (also known as HEF-1), calmodulin or PIFO; or interaction with inhibitory proteins, such as TCHP [7] , [8] , [9] , [10] . However, the mechanisms regulating cilia disassembly are not yet understood in great detail. Notably, whether the interaction between AURKA and HDAC6 is regulated has not been addressed. The MST1/2-SAV1 complex is a core component of the Hippo pathway [11] , [12] . MST1 and MST2 are serine/threonine kinases with redundant functions whose activities are enhanced by interaction with the SAV1 scaffold protein. In the context of the Hippo pathway, the MST1/2-SAV1 complex activates its downstream kinase(s) LATS1/2, which, in turn, inhibits the oncogenic transcriptional co-activators YAP and TAZ. The Hippo pathway is activated by epithelial cell polarity; however, whether the components of this pathway contribute to cell polarity processes has not been investigated. In T cells, MST1 supports polarized trafficking of endosomes towards the immune synapse [13] ; however, it is not known whether it performs a similar role in epithelial cells. In addition to their role in the Hippo pathway, MST1/2 also has a noncanonical function: regulation of microtubule stability/dynamics. For example, loss of MST1/2 or its target(s) NDR1/2 destabilizes kinetochore-microtubule attachment during mitosis [14] , [15] . Hippo (homologue of MST1/2) or Ndr Drosophila mutants exhibit a collapsed dendrite network in the brain [16] . Given these results and the fact that primary cilia—which are built from microtubules—are also downstream of cell polarity [17] , we sought to determine whether MST1/2-SAV1 regulates ciliogenesis. In this study, we show that MST1 is activated during ciliogenesis and localizes to the basal body of cilia. Depletion of MST1/2 or SAV1 impairs ciliogenesis in cultured cells and induces ciliopathy phenotypes in zebrafish. MST1/2-SAV1 regulates ciliogenesis through two independent mechanisms: (1) MST1/2 binds and phosphorylates AURKA, leading to dissociation of the AURKA/HDAC6 cilia-disassembly complex; and (2) MST1/2-SAV1 associates with the NPHP transition-zone complex, promoting ciliary localization of multiple ciliary cargoes. Our results suggest that components of the Hippo pathway contribute to establish a polarized cell structure in addition to regulating proliferation. MST1/2-SAV1 localization and activation in ciliated cells As the first step in our investigation of the role of MST1/2 and SAV1 in ciliogenesis, we examined the localizations of these proteins in ciliated cells. In cultured cells, ciliogenesis is induced by serum starvation of cells in a confluent monolayer. In retinal pigment epithelial (RPE) cells, green fluorescent protein (GFP)-fused SAV1 was found at the centrosome of proliferating cells and at the basal body of ciliated cells ( Fig. 1a ). Immunostaining with an antibody against T183-phosphorylated MST1, the active form, revealed that activated MST1 was localized to the basal body in ciliated cells but was not detectable in proliferating cells ( Fig. 1b ). The specificity of the immunostaining was confirmed by small interfering RNA (siRNA)-mediated depletion of MST1/2. Examination of total MST1 localization by hemagglutinin (HA) immunostaining in RPE cells expressing HA-MST1 revealed that MST1 was diffusely localized throughout the cytoplasm both in proliferating and ciliated cells ( Supplementary Fig. 1 ). This indicates that a subpopulation of MST1 is specifically activated in cilia. Western blot analysis also showed that MST1/2 was more active in ciliated cells as indicated by increased T183-phosphorylated MST1 and T35-phosphorylated MOB1, an established substrate of MST1/2 (ref. 18 ; Fig. 1c ). To generalize these findings, we also examined mIMCD3 cells (a murine inner medullary collecting duct cell line). Similar to RPE, GFP-SAV1 was found at both centrosome and basal body of cilia ( Supplementary Fig. 2a ) in mIMCD3 cells. Immunofluorescence signal of activated MST1 was much weaker in mIMCD3 than in RPE. Nevertheless, ~20–30% of ciliated cells had activated MST1 signal in the basal body, which was not detectable in either proliferating cells or Mst1/2-depleted serum-starved cells ( Supplementary Fig. 2b ). Phosphorylated Mst1 and Mob1 also increased in ciliated mIMCD3 cells as judged by western blot analysis ( Supplementary Fig. 2c ). These results suggest a possible role for MST1/2 and SAV1 in ciliogenesis. 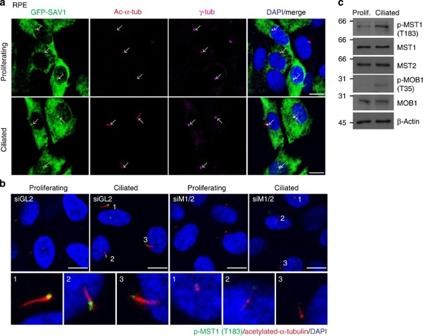Figure 1: MST1 is activated during ciliogenesis and localizes to the basal body of cilia together with SAV1. (a) Proliferating or ciliated RPE cells transduced with GFP-SAV1 were immunostained for GFP, acetylated α-tubulin, γ-tubulin and counterstained with 4′,6-diamidino-2-phenylindole (DAPI). Arrows indicate co-localized signals. (b) Proliferating or ciliated RPE cells transfected with control or MST1/2 siRNA were immunostained for T183-phosphorylated (active) MST1 (p-MST1 (T183)), acetylated α-tubulin and counterstained with DAPI. Below are enlarged images of indicated cells. Scale bars ina,b, 10 μm. (c) Extracts of proliferating or ciliated RPE cells were fractionated by SDS–PAGE and immunoblotted with the indicated antibodies. We performed all experiments three times independently and obtained similar results. Figure 1: MST1 is activated during ciliogenesis and localizes to the basal body of cilia together with SAV1. ( a ) Proliferating or ciliated RPE cells transduced with GFP-SAV1 were immunostained for GFP, acetylated α-tubulin, γ-tubulin and counterstained with 4′,6-diamidino-2-phenylindole (DAPI). Arrows indicate co-localized signals. ( b ) Proliferating or ciliated RPE cells transfected with control or MST1/2 siRNA were immunostained for T183-phosphorylated (active) MST1 (p-MST1 (T183)), acetylated α-tubulin and counterstained with DAPI. Below are enlarged images of indicated cells. Scale bars in a , b , 10 μm. ( c ) Extracts of proliferating or ciliated RPE cells were fractionated by SDS–PAGE and immunoblotted with the indicated antibodies. We performed all experiments three times independently and obtained similar results. Full size image Depletion of MST1/2 or SAV1 impairs ciliogenesis To test whether MST1/2 or SAV1 regulates ciliogenesis, we depleted MST1/2 or SAV1 in RPE cells with siRNA ( Fig. 2a ). Cells depleted of MST1/2 or SAV1 had a reduced number of ciliated cells and the lengths of the remaining cilia were shorter ( Fig. 2b–d ). Impaired ciliogenesis was also observed in mIMCD3 cells depleted of Mst1/2 or Sav1 ( Supplementary Fig. 3 ). In Mst1/2-depleted mIMCD3 cells stably expressing Mst1/2 short-hairpin RNA (shRNA), reconstitution with human MST1 wild-type (MST1 WT) rescued ciliogenesis, whereas a kinase dead (KD) MST1 mutant (MST1 KD) did not ( Fig. 2g ). MST1 WT and KD proteins were expressed at comparable levels but only MST1 WT-reconstituted cells restored Mob1 phosphorylation ( Fig. 2e ). Similarly, reconstitution of Sav1-depleted mIMCD3 cells with SAV1 WT or a ΔWW mutant rescued ciliogenesis; however, reconstitution with the SAV1 ΔSARAH mutant, which is unable to interact with MST1/2, failed to do so ( Fig. 2h , see Fig. 7e for domain map of SAV1). We confirmed that rescued SAV1 proteins were expressed at comparable levels and that only SAV1 WT- and ΔWW-reconstituted cells restored interaction with MST1 ( Fig. 2f ). Thus, these reconstitution experiments exclude the possibility of off-target effects and indicate that the MST1/2-SAV1 complex is required for ciliogenesis in a kinase activity-dependent manner. Co-depletion of MST1/2 and SAV1 in RPE cells did not further impair ciliogenesis compared with depletion of individual components alone ( Supplementary Fig. 4 ). This again suggests that MST1/2 and SAV1 majorly function together during ciliogenesis, although their independent functions cannot be perfectly ruled out. We also found that the percentage of Mst1/2-null mouse embryonic fibroblasts (MEFs) containing cilia was reduced (Control, 54.75%; Mst1/2-null 28.01%). 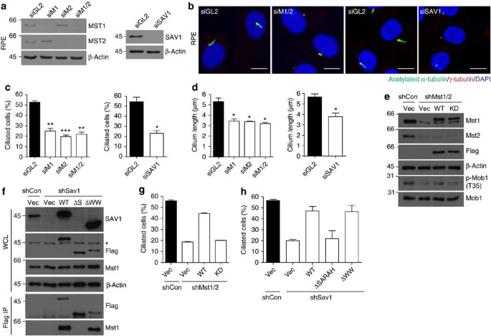Figure 2: Depletion of MST1/2 and SAV1 impairs ciliogenesis in cultured cells. (a) Knockdown of MST1/2 and SAV1 in RPE cells was confirmed with western blotting. (b) Representative images of ciliated RPE cells treated with the indicated siRNAs. Scale bar, 10 μm. (c,d) Frequencies of ciliated cells and lengths of cilia were quantified in the indicated samples. (e) mIMCD3 cells stably expressing shRNA against Mst1/2 were reconstituted with empty vector, Flag-MST1 WT or Flag-MST1 KD. Cell extracts were immunoblotted with the indicated antibodies. (f) Similar to (e), mIMCD3 cells stably expressing shRNA against Sav1 were reconstituted with empty vector, Flag-SAV1 WT, Flag-SAV1 ΔSARAH or Flag-SAV1 ΔWW. Cell extracts were immunoblotted with the indicated antibodies. One milligram of extracts was immunoprecipitated with an anti-Flag antibody and immunoblotted to detect endogenous co-purified Mst1. Note that SAV1 antibody does not detect Flag-SAV1 ΔSARAH because the antibody detects C-terminal part of SAV1 protein. WCL, whole cell lysates. *, nonspecific band. (g) Frequencies of ciliated cells inewere quantified. (h) Frequencies of ciliated cells infwere quantified. Error bars inc,dindicate s.e.m.’s of three independent experiments (*P<0.05, **P<0.01, ***P<0.001; Student’st-test). Forg,h, two biological replicates were performed. At least 200 cells from four to five random fields per slide were counted. Figure 2: Depletion of MST1/2 and SAV1 impairs ciliogenesis in cultured cells. ( a ) Knockdown of MST1/2 and SAV1 in RPE cells was confirmed with western blotting. ( b ) Representative images of ciliated RPE cells treated with the indicated siRNAs. Scale bar, 10 μm. ( c , d ) Frequencies of ciliated cells and lengths of cilia were quantified in the indicated samples. ( e ) mIMCD3 cells stably expressing shRNA against Mst1/2 were reconstituted with empty vector, Flag-MST1 WT or Flag-MST1 KD. Cell extracts were immunoblotted with the indicated antibodies. ( f ) Similar to ( e ), mIMCD3 cells stably expressing shRNA against Sav1 were reconstituted with empty vector, Flag-SAV1 WT, Flag-SAV1 ΔSARAH or Flag-SAV1 ΔWW. Cell extracts were immunoblotted with the indicated antibodies. One milligram of extracts was immunoprecipitated with an anti-Flag antibody and immunoblotted to detect endogenous co-purified Mst1. Note that SAV1 antibody does not detect Flag-SAV1 ΔSARAH because the antibody detects C-terminal part of SAV1 protein. WCL, whole cell lysates. *, nonspecific band. ( g ) Frequencies of ciliated cells in e were quantified. ( h ) Frequencies of ciliated cells in f were quantified. Error bars in c , d indicate s.e.m.’s of three independent experiments (* P <0.05, ** P <0.01, *** P <0.001; Student’s t -test). For g , h , two biological replicates were performed. At least 200 cells from four to five random fields per slide were counted. Full size image Figure 7: MST1/2–SAV1 forms a complex with NPHP1. ( a ) 293T cells were transfected with Flag-NPHP1/4/8 and HA-SAV1 or HA-MST1. Flag-NPHP was immunoprecipitated and immunoprecipitates were examined for the presence of HA-MST1 or HA-SAV1. *, heavy chain. 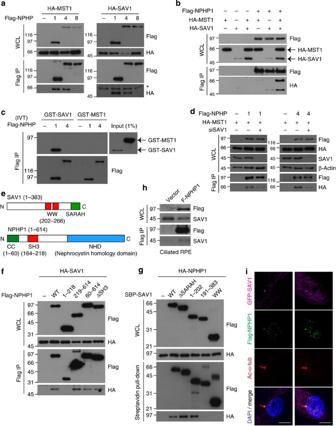Figure 7: MST1/2–SAV1 forms a complex with NPHP1. (a) 293T cells were transfected with Flag-NPHP1/4/8 and HA-SAV1 or HA-MST1. Flag-NPHP was immunoprecipitated and immunoprecipitates were examined for the presence of HA-MST1 or HA-SAV1. *, heavy chain. (b) 293T cells were transfected as indicated and complex formation was examined with the help of co-immunoprecipitation. (c) Purified recombinant GST-SAV1 or GST-MST1 protein was incubated within vitro-translated(IVT) Flag-NPHP1 or Flag-NPHP4 followed by immunoprecipitation with an anti-Flag antibody. (d) 293T cells were transfected with control or SAV1 siRNA. One day after siRNA transfection, cells were transfected with indicated combinations of DNA. Co-immunoprecipitation was performed as indicated. (e) Domain architecture of SAV1 and NPHP1. (f) Interaction mapping of HA-SAV1 and Flag-NPHP1 truncation mutants. (g) Interaction mapping of HA-NPHP1 and SBP–SAV1 truncation mutants. (h) RPE cells transduced with control or Flag-NPHP1 were immunoprecipitated with an anti-Flag antibody. Endogenous SAV1 was co-purified with Flag-NPHP1. (i) RPE cells were transduced with Flag-NPHP1 and GFP-SAV1. After ciliogenesis induction, cells were immunostained with antibodies against Flag, GFP and acetylated α-tubulin, and counterstained with DAPI. Scale bar, 10 μm. We performed all experiments three times independently and obtained similar results. ( b ) 293T cells were transfected as indicated and complex formation was examined with the help of co-immunoprecipitation. ( c ) Purified recombinant GST-SAV1 or GST-MST1 protein was incubated with in vitro-translated (IVT) Flag-NPHP1 or Flag-NPHP4 followed by immunoprecipitation with an anti-Flag antibody. ( d ) 293T cells were transfected with control or SAV1 siRNA. One day after siRNA transfection, cells were transfected with indicated combinations of DNA. Co-immunoprecipitation was performed as indicated. ( e ) Domain architecture of SAV1 and NPHP1. ( f ) Interaction mapping of HA-SAV1 and Flag-NPHP1 truncation mutants. ( g ) Interaction mapping of HA-NPHP1 and SBP–SAV1 truncation mutants. ( h ) RPE cells transduced with control or Flag-NPHP1 were immunoprecipitated with an anti-Flag antibody. Endogenous SAV1 was co-purified with Flag-NPHP1. ( i ) RPE cells were transduced with Flag-NPHP1 and GFP-SAV1. After ciliogenesis induction, cells were immunostained with antibodies against Flag, GFP and acetylated α-tubulin, and counterstained with DAPI. Scale bar, 10 μm. We performed all experiments three times independently and obtained similar results. Full size image In response to apoptotic stimuli, MST1/2 is cleaved by caspase-3 and the N-terminal fragment containing the kinase domain translocates into the nucleus [19] . Cleaved MST1 promotes cell death in part by phosphorylating H2B on S14 (refs 20 , 21 ). In our experimental condition, neither RPE nor mIMCD3 cells showed noticeable cell death in response to serum starvation. Furthermore, activated MST1 was found at the basal body in ciliated cells. Therefore, it is unlikely that the cleaved form of MST1 plays a role in ciliogenesis. However, it still remains possible that undetectable amount of cleaved MST1 is functionally important. To examine this possibility, we reconstituted shMst1/2-expressing mIMCD3 cells with either MST1 WT or MST1 D326/349N mutant, a caspase cleavage-resistant form [22] , [23] . Both WT and D326/349N mutant restored ciliogenesis and Mob1 phosphorylation to comparable levels ( Supplementary Fig. 5 ). Thus, we conclude that MST1/2 functions as full-length proteins during ciliogenesis. Normal ciliogenesis in the absence of LATS1/2 or YAP In the canonical Hippo pathway, the MST1/2-SAV1 complex regulates LATS1/2, which, in turn, inhibits the YAP activity. Thus, we examined the requirements of these components of the Hippo pathway in ciliogenesis of RPE cells. To this end, we depleted LATS1/2 and YAP using siRNA. In contrast to MST1/2-SAV1 depletion, loss of these downstream components did not cause ciliogenesis impairment, ruling out the role of the canonical Hippo pathway in ciliogenesis ( Fig. 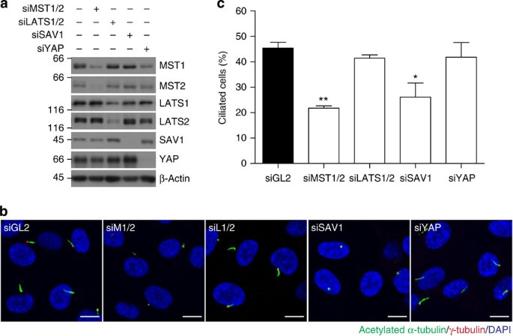3 ). Figure 3: LATS1/2 and YAP are dispensable for ciliogenesis. (a) RPE cells were transfected with indicated siRNAs. Gene knockdown was confirmed with western blot analysis. (b) Representative images fora. Scale bar, 10 μm. (c) Frequencies of ciliated cells froma,bwere quantified. Error bars incindicate s.e.m.’s of three independent experiments (*P<0.05, **P<0.01; Student’st-test). At least 200 cells from four to five random fields per slide were counted. Figure 3: LATS1/2 and YAP are dispensable for ciliogenesis. ( a ) RPE cells were transfected with indicated siRNAs. Gene knockdown was confirmed with western blot analysis. ( b ) Representative images for a . Scale bar, 10 μm. ( c ) Frequencies of ciliated cells from a , b were quantified. Error bars in c indicate s.e.m.’s of three independent experiments (* P <0.05, ** P <0.01; Student’s t -test). At least 200 cells from four to five random fields per slide were counted. Full size image Normal contact inhibition in the absence of MST1/2 or SAV1 Serum starvation-induced ciliogenesis requires contact inhibition and cell-cycle exit. Upon induction of ciliogenesis, cells depleted of MST1/2 or SAV1 showed a reduction in the number of cells positive for the proliferation marker, Ki67, that was comparable to that of control cells ( Supplementary Fig. 6a ). Thus, it is unlikely that the ciliogenesis defects of MST1/2- or SAV1-depleted cells are attributable to secondary effects of a defect in cell-cycle exit. Since the Hippo pathway was originally suggested to mediate cell contact inhibition [24] , we further examined contact inhibition in MST1/2- or SAV1-depleted cells. Cells depleted of MST1/2 or SAV1 exhibited a normal reduction in 5-bromodeoxyuridine (BrdU) uptake (marker of proliferation) as their cell density increased ( Supplementary Fig. 6b ). Moreover, the induction of phosphorylation of YAP and p27, established markers of contact inhibition, was similar in these cells and control cells ( Supplementary Fig. 6c ). Collectively, these observations suggest that MST1/2 and SAV1 are not involved in contact inhibition, a result that is fully consistent with a number of recent studies in cell culture systems [25] , [26] , [27] , [28] , [29] . Mst1/2 or Sav1 depletion abrogates acini formation Next, we performed functional assays of primary cilia. Loss of ciliogenesis genes often abrogates the acinar architecture of epithelial cells in three-dimensional (3D) cultures [30] . Therefore, we examined acini development in Mst1/2- or Sav1-depleted mIMCD3 cells. Indeed, in the absence of Mst1/2 or Sav1, most acini showed a collapsed lumen without cilia formation, whereas only 10% of control acini showed mild abnormalities ( Fig. 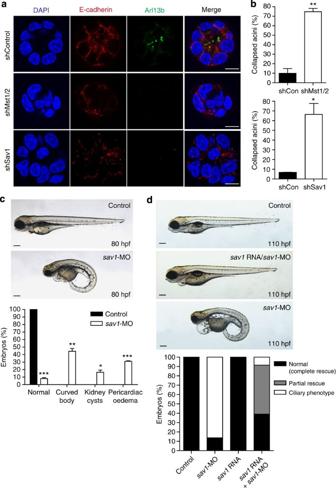4a,b ). Figure 4: Depletion of MST1/2 and SAV1 abrogates 3D acini architecture and induces ciliopathy phenotypes in zebrafish. (a) mIMCD3 cells stably expressing shRNAs targeting Mst1/2 or Sav1 were cultured in 3D for 4 days to induce acini formation. Acini were immunostained for Arl13b and E-cadherin, and counterstained with DAPI. A total of 15 sections between the bottom and top of acini were imaged by confocal microscopy; representative images from the middle point are shown. Scale bar, 10 μm. (b) Acini fromawith collapsed lumen were quantified. Error bars indicate s.e.m.’s of three independent experiments. At least 20 acini per slide were imaged and quantified (*P<0.05, **P<0.01; Student’st-test). (c) Knockdown ofsav1leads to a curved-tail defect, cardiac oedema and cystic kidney.Upper:Control embryos at 80 h post fertilization (hpf).Middle: Sav1morphants exhibited multiple ciliopathy phenotypes compared with control embryos.Bottom:Quantification of embryos with the indicated ciliopathy phenotypes in control andsav1morphants. Error bars indicate s.e.m.’s of three independent experiments. At least 100 embryos were injected for each independent experiment. (*P<0.05, **P<0.01, ***P<0.001; Student’st-test). (d) Rescue ofsav1morphant phenotypes by co-injection ofsav1-RNA at 110 hpf.Top-most:Control embryos;second:rescue of ciliopathy phenotypes insav1morphants by injection of 50 pgsav1mRNA; third:sav1morphant embryos; bottom: frequency of ciliopathy phenotypes in each treatment group. Co-injection ofsav1mRNA andsav1morpholino rescued the morphant phenotypes. Controln=78,sav1-MOn=80,sav1-RNAn=71 andsav1-RNA+sav1-MOn=82. Scale bar, 0.2 mm. Figure 4: Depletion of MST1/2 and SAV1 abrogates 3D acini architecture and induces ciliopathy phenotypes in zebrafish. ( a ) mIMCD3 cells stably expressing shRNAs targeting Mst1/2 or Sav1 were cultured in 3D for 4 days to induce acini formation. Acini were immunostained for Arl13b and E-cadherin, and counterstained with DAPI. A total of 15 sections between the bottom and top of acini were imaged by confocal microscopy; representative images from the middle point are shown. Scale bar, 10 μm. ( b ) Acini from a with collapsed lumen were quantified. Error bars indicate s.e.m.’s of three independent experiments. At least 20 acini per slide were imaged and quantified (* P <0.05, ** P <0.01; Student’s t -test). ( c ) Knockdown of sav1 leads to a curved-tail defect, cardiac oedema and cystic kidney. Upper: Control embryos at 80 h post fertilization (hpf). Middle: Sav1 morphants exhibited multiple ciliopathy phenotypes compared with control embryos. Bottom: Quantification of embryos with the indicated ciliopathy phenotypes in control and sav1 morphants. Error bars indicate s.e.m.’s of three independent experiments. At least 100 embryos were injected for each independent experiment. (* P <0.05, ** P <0.01, *** P <0.001; Student’s t -test). ( d ) Rescue of sav1 morphant phenotypes by co-injection of sav1 -RNA at 110 hpf. Top-most: Control embryos; second: rescue of ciliopathy phenotypes in sav1 morphants by injection of 50 pg sav1 mRNA; third: sav1 morphant embryos; bottom: frequency of ciliopathy phenotypes in each treatment group. Co-injection of sav1 mRNA and sav1 morpholino rescued the morphant phenotypes. Control n =78, sav1 -MO n =80, sav1 -RNA n =71 and sav1 -RNA+ sav1 -MO n =82. Scale bar, 0.2 mm. Full size image Sav1 depletion induces ciliopathy phenotypes in zebrafish To further examine the requirement for the MST1/2-SAV1 complex in vivo , we utilized a zebrafish model, injecting antisense morpholinos against zebrafish sav1 . The efficacy of morpholino-mediated knockdown was confirmed using a sav1 -EGFP construct ( Supplementary Fig. 7 ). Notably, depletion of sav1 induced several ciliopathy phenotypes ( Fig. 4c,d ). Roughly, half of sav1 morphants exhibited a curved-body axis and cardiac oedema ( Fig. 4c ), and about one quarter of sav1 morphants displayed mild-to-severe cystic kidney, which is a typical ciliopathy phenotype ( Fig. 4c ). However, left–right asymmetry and heart looping appeared normal in sav1 morphants, possibly due to maternal effects (data not shown). Acetylated α-tubulin staining further showed that sav1 morphants had scarce and shorter cilia in the pronephric ducts compared with controls ( Supplementary Fig. 8 ). Importantly, co-injection of sav1 mRNA rescued the ciliopathy phenotypes of sav1 morphants, confirming the specificity of the morpholino ( Fig. 4d ). Intriguingly, we could not identify a homologue of MST1 in the zebrafish genome. An MST2 homologue-only morphant showed no obvious phenotype (data not shown), suggesting the possible existence of an as yet uncharacterized functional homologue of MST1 in zebrafish. MST1/2-SAV1 loss triggers AURKA-dependent cilia disassembly Next, we attempted to understand the mechanism by which MST1/2-SAV1 regulates ciliogenesis. One possibility is that loss of MST1/2-SAV1 destabilizes cilia and triggers cilia disassembly. Two observations prompted us to pursue this hypothesis. First, depletion of MST1/2 or SAV1 after serum starvation led to the disappearance of pre-established cilia, indicating that MST1/2-SAV1 is required for cilia maintenance ( Fig. 5a ). The other supporting evidence was obtained from a gain-of-function study. By clonal selection after HA-MST1 transfection, we established cell lines that overexpressed MST1 by approximately twofold compared with the endogenous level ( Fig. 5b ). These clones had about twofold increase in phosphorylated MOB1 ( Fig. 5b ) and MST1-SAV1 complex ( Fig. 5c ). At this expression level, MST1 did not induce cell death (data not shown), and there was no difference in basal ciliogenesis index in these cells upon serum starvation ( Fig. 5d ). However, following serum re-stimulation, cilia disassembly was markedly attenuated in cells with increased MST1 expression ( Fig. 5d ). Subsequent G1/S progression requires cilia disassembly [31] , [32] . Consistent with the delayed cilia disassembly phenotype, cells with increased MST1 expression exhibited significantly attenuated G1/S progression, as determined by EdU-incorporation assays and western blot analysis for cell-cycle markers ( Supplementary Fig. 9 ). 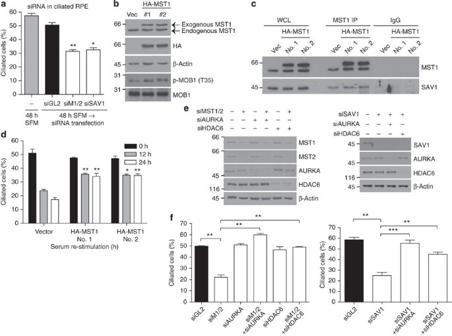These results suggest that MST1/2-SAV1 contributes to cilia maintenance by antagonizing the cilia-disassembly pathway. Figure 5: Depletion of MST1/2 and SAV1 triggers AURKA/HDAC6-mediated cilia disassembly. (a) Ciliated RPE cells were transfected with the indicated siRNAs. Two technical replicates were fixed before transfection. Two days after transfection, cells were fixed and immunostained. Frequencies of remaining cilia were quantified. SFM, serum-free media. (b) RPE cells stably expressing HA-MST1 were established by clonal selection. Near-endogenous expression of MST1 was confirmed in two clones. Endogenous and HA-tagged exogenous MST1 are indicated. Notably, phospho-MOB1 was also increased about twofold in HA-MST1-expressing cells. (c) Protein extracts of cells frombwere immunoprecipitated with an anti-MST1 antibody. Co-purified endogenous SAV1 was detected with western blot analysis. In HA-MST1-expressing cells, the MST1–SAV1 complex was increased about twofold. (d) Ciliogenesis was induced in control and HA-MST1-expressing cells followed by serum re-stimulation. Frequencies of ciliated cells were quantified at the indicated time points after serum re-addition. (e) RPE cells were transfected with the indicated siRNA combinations. Gene knockdown was confirmed with western blot analysis. (f) Frequencies of ciliated cells were quantified frome. Error bars ina,d,findicate s.e.m.’s of three independent experiments (*P<0.05, **P<0.01, ***P<0.001; Student’st-test). Ford, each HA-MST1 clones were compared with control cells at given time points. At least 200 cells from four to five random fields per slide were counted. Figure 5: Depletion of MST1/2 and SAV1 triggers AURKA/HDAC6-mediated cilia disassembly. ( a ) Ciliated RPE cells were transfected with the indicated siRNAs. Two technical replicates were fixed before transfection. Two days after transfection, cells were fixed and immunostained. Frequencies of remaining cilia were quantified. SFM, serum-free media. ( b ) RPE cells stably expressing HA-MST1 were established by clonal selection. Near-endogenous expression of MST1 was confirmed in two clones. Endogenous and HA-tagged exogenous MST1 are indicated. Notably, phospho-MOB1 was also increased about twofold in HA-MST1-expressing cells. ( c ) Protein extracts of cells from b were immunoprecipitated with an anti-MST1 antibody. Co-purified endogenous SAV1 was detected with western blot analysis. In HA-MST1-expressing cells, the MST1–SAV1 complex was increased about twofold. ( d ) Ciliogenesis was induced in control and HA-MST1-expressing cells followed by serum re-stimulation. Frequencies of ciliated cells were quantified at the indicated time points after serum re-addition. ( e ) RPE cells were transfected with the indicated siRNA combinations. Gene knockdown was confirmed with western blot analysis. ( f ) Frequencies of ciliated cells were quantified from e . Error bars in a , d , f indicate s.e.m.’s of three independent experiments (* P <0.05, ** P <0.01, *** P <0.001; Student’s t -test). For d , each HA-MST1 clones were compared with control cells at given time points. At least 200 cells from four to five random fields per slide were counted. Full size image AURKA and its target HDAC6 have been proposed to mediate cilia disassembly upon cell-cycle re-entry [7] . Upon receiving a cue for cell-cycle re-entry, AURKA phosphorylates and activates HDAC6, which in turn deacetylates ciliary tubulins. Therefore, we asked whether this pathway was responsible for the phenotype induced by depletion of MST1/2 or SAV1. Remarkably, co-depletion of AURKA or HDAC6 restored ciliogenesis in MST1/2-SAV1-depleted cells ( Fig. 5e,f ), indicating that on-going AURKA/HDAC6-mediated cilia disassembly is the cause for the observed phenotype. MST1 dissociates the AURKA/HDAC6 cilia-disassembly complex To obtain further mechanistic insight, we examined the interaction between MST1/2 and AURKA. MST1 interacted with AURKA in both cultured cells and under cell-free ( in vitro ) conditions ( Supplementary Fig. 10a,b ). In addition, purified MST1 phosphorylated full-length AURKA in vitro ( Fig. 6a ). We then tested whether MST1/2 directly affects the kinase activity of AURKA. However, we could not detect any significantly elevated kinase activity of AURKA immunoprecipitated from MST1/2-SAV1-depleted cells. Moreover, pre-incubation of recombinant AURKA with purified MST1 did not reduce AURKA activity (data not shown). We next attempted to determine the phosphorylation site(s) on AURKA by MST1/2. We first divided AURKA into N-terminal fragment (preceding kinase domain, amino acids 1–130) and C-terminal fragment (amino acids 131–403). MST1 preferentially phosphorylated N-terminal portion of AURKA ( Supplementary Fig. 10c ). Then, we mutated eight evolutionarily conserved serine or threonine residues among human, mouse and rat within the N-terminal part of AURKA to alanine. However, all these mutant proteins were still phosphorylated by MST1 in vitro ( Supplementary Fig. 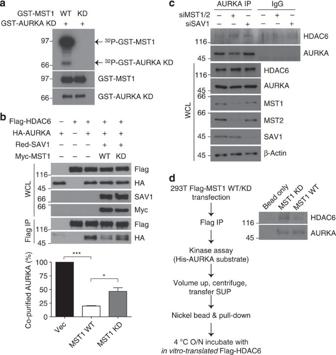10d ), suggesting that multiple sites in AURKA can be phosphorylated or that the target site(s) in AURKA is flexible so that mutating one target site might give rise to phosphorylation at alternative site(s). Figure 6: MST1 dissociates the AURKA/HDAC6 complex by phosphorylating AURKA. (a) MST1 phosphorylates AURKAin vitro. The recombinant GST-MST1 protein was incubated with GST-AURKA and γ-32P-labelled ATP for 30 min. Reaction products were analysed by autoradiography and western blot analysis. (b) 293T cells were transfected with the indicated constructs. Two days after transfection, the interaction between AURKA and HDAC6 was examined by co-immunoprecipitation. The amount of co-purified AURKA was quantified using the Image J programme. Error bars indicate s.e.m.’s of three independent experiments (*P<0.05, ***P<0.001; Student’st-test). (c) Ciliated RPE cells were transfected with the indicated siRNAs. Two days after transfection, the interaction between AURKA and HDAC6 was examined with immunoprecipitation of endogenous AURKA. (d)Left:Schematic depiction ofin vitrobinding assay procedures. Flag-MST1 WT or Flag-MST1 KD was immunoprecipitated from 293T cells and used to phosphorylate recombinant His-AURKA protein with cold ATP. Flag-MST1 was washed out and His-AURKA was incubated within vitro-translated Flag-HDAC6.Right:Results ofin vitrobinding assays. Pre-incubation with MST1 WT reduced AURKA/HDAC6 complex formation. We performed all experiments three times independently and obtained similar results. Figure 6: MST1 dissociates the AURKA/HDAC6 complex by phosphorylating AURKA. ( a ) MST1 phosphorylates AURKA in vitro . The recombinant GST-MST1 protein was incubated with GST-AURKA and γ- 32 P-labelled ATP for 30 min. Reaction products were analysed by autoradiography and western blot analysis. ( b ) 293T cells were transfected with the indicated constructs. Two days after transfection, the interaction between AURKA and HDAC6 was examined by co-immunoprecipitation. The amount of co-purified AURKA was quantified using the Image J programme. Error bars indicate s.e.m.’s of three independent experiments (* P <0.05, *** P <0.001; Student’s t -test). ( c ) Ciliated RPE cells were transfected with the indicated siRNAs. Two days after transfection, the interaction between AURKA and HDAC6 was examined with immunoprecipitation of endogenous AURKA. ( d ) Left: Schematic depiction of in vitro binding assay procedures. Flag-MST1 WT or Flag-MST1 KD was immunoprecipitated from 293T cells and used to phosphorylate recombinant His-AURKA protein with cold ATP. Flag-MST1 was washed out and His-AURKA was incubated with in vitro- translated Flag-HDAC6. Right: Results of in vitro binding assays. Pre-incubation with MST1 WT reduced AURKA/HDAC6 complex formation. We performed all experiments three times independently and obtained similar results. Full size image We next tested whether MST1 affected the interaction between AURKA and its effector HDAC6. Intriguingly, MST1 overexpression reduced the interaction between AURKA and HDAC6 in an MST1 kinase activity-dependent manner ( Fig. 6b ). More importantly, depletion of MST1/2 or SAV1 in ciliated RPE cells increased AURKA/HDAC6 complex formation ( Fig. 6c ). Last, we directly addressed the role of MST1 in interfering with AURKA/HDAC6 complex formation in vitro . AURKA pre-incubated with MST1 WT, but not with an MST1 KD mutant, showed reduced binding to purified HDAC6 ( Fig. 6d ). Collectively, these data suggest that MST1/2 interferes with formation of the AURKA/HDAC6 cilia-disassembly complex. MST1/2-SAV1 interacts with the NPHP transition-zone complex The transition zone of primary cilia regulates ciliary composition [33] , [34] . Two main transition-zone complexes are known: the NPHP1/4/8 complex and the Tectonic complex [35] , [36] , [37] . Interestingly, a previous proteomic study identified MST2, SAV1 and TAO kinase, a recently identified activator of MST1/2 (refs 38 , 39 ), as potential binding partners of the NPHP complex [30] . Moreover, MST1 promotes polarized trafficking of β1-integrin endosomes towards the immune synapse in T cells [13] . Given the potential interaction with the NPHP complex and the suggested function of MST1 in regulating polarized trafficking, we postulated that MST1/2 and SAV1 function as components of the NPHP complex. Of note, depletion of TAO1 or TAO3 also impaired ciliogenesis in serum-starved RPE cells ( Supplementary Fig. 11 ). Although Habbig et al. [40] reported no interaction between MST1 and NPHP1/4, in our hands, a co-immunoprecipitation study showed that MST1 and SAV1 clearly associated with NPHP components, especially with NPHP1 and NPHP4 ( Fig. 7a ). Reason for this discrepancy is unclear yet; however, it might be because of different experimental conditions or different NPHP splicing variants used in the interaction assays. SAV1 interacted more strongly with NPHP1/4 than did MST1 ( Fig. 7b and data not shown). Importantly, co-expression of MST1 and SAV1 dramatically increased the interaction between MST1 and NPHP1/4 ( Fig. 7b and data not shown), indicating that SAV1 acts as a scaffold for MST1 and NPHP1/4. Co-expression of MST1 increased SAV1 stability in this experiment, as reported before [41] . An in vitro binding assay using purified recombinant GST-SAV1, GST-MST1 and in vitro- translated Flag-NPHP1/4 showed that only NPHP1 strongly pulled down SAV1, whereas GST-MST1 did not interact with either NPHP components ( Fig. 7c ). It is important to note that NPHP4 acts as a scaffold for NPHP1/8, and NPHP1 and -8 do not interact directly in vitro [30] , which is in line with our data. To definitely confirm the idea that SAV1 scaffolds MST1 and NPHP1/4, we performed co-immunoprecipitation of MST1 and NPHP1/4 in SAV1-depleted cells. In the absence of SAV1, the interaction between MST1 and NPHP1/4 substantially decreased ( Fig. 7d ). As expected, depletion of NPHP4 did not affect the interaction between SAV1 and NPHP1 ( Supplementary Fig. 12c ). In contrast, depletion of NPHP1 substantially decreased the interaction between SAV1 and NPHP4 ( Supplementary Fig. 12b ). We next identified the domains responsible for the NPHP1–SAV1 interaction using deletion mutants. The nephrocystin homology domain of NPHP1 was required and sufficient for the interaction with SAV1 ( Fig. 7e,f ). Regions N terminal to the WW domain of SAV1 were most critical for binding to NPHP1 ( Fig. 7e,g ). Importantly, Flag-NPHP1 co-immunoprecipitated endogenous SAV1 in ciliated RPE cells ( Fig. 7h ), and co-immunostaining confirmed that their interaction occurred at the base of cilia ( Fig. 7i ). We conclude that SAV1 associates through its N-terminal region with the NPHP transition-zone complex, directly contacting the NPHP1 nephrocystin homology domain region, and thereby recruits MST1/2. MST1/2-SAV1 regulates localization of ciliary proteins Having established the interaction between MST1/2–SAV1 and the NPHP complex, we tested whether the loss of MST1/2-SAV1 affects localization of ciliary proteins. To this end, we have examined four ciliary proteins: Rab8a, Smo, RPGR and Arl13b. Depletion of MST1/2 or SAV1 reduced ciliary localization of these cargoes to varying degrees, except for Arl13b ( Fig. 8a–d ). The reason why Arl13b localization is unaffected by MST1/2–SAV1 depletion is unclear yet. Possibly, Arl13b is majorly transported via NPHP-independent routes. Of note, Arl13b localization was significantly impaired in cells depleted of the Tectonic complex [35] . Importantly, depletion of MST1/2 or SAV1 in an AURKA-co-depleted background rescued ciliogenesis ( Fig. 5f ) but still reduced ciliary localization of Rab8a and RPGR ( Fig. 8e,f ). This indicates that the MST1/2–SAV1 complex also regulates ciliary localization of these proteins independent of AURKA/HDAC6. Last, if the MST1/2–SAV1 complex functions by interacting with NPHP1, one would expect that co-depletion of NPHP1 and MST1/2–SAV1 would not further enhance the phenotype. Indeed, the impact of co-depleting NPHP1 and MST1/2 or SAV1 on ciliary localization of Rab8a and RPGR was comparable to depletion of NPHP1 alone ( Supplementary Fig. 13 ). 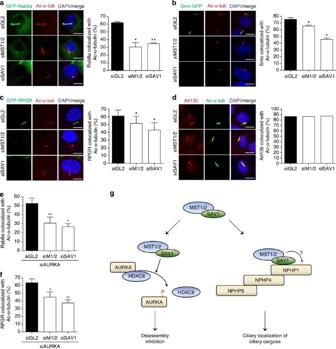Figure 8: Depletion of MST1/2 and SAV1 impairs ciliary localization of ciliary proteins. (a–d) RPE cells were transduced with GFP-Rab8a (a), Smo-GFP (b) or GFP-RPGR (c). Each cell type was transfected with siRNA against MST1/2 or SAV1, and ciliogenesis was induced. Cells were co-immunostained for GFP (a–c) or Arl13b (d) and acetylated α- and γ-tubulin. γ-tubulin staining is presented only in merged images. Scale bar, 10 μm. (e,f) Ciliary localization indexes for Rab8a and RPGR were measured in AURKA and MST1/2-SAV1 co-depleted backgrounds. Error bars indicate s.e.m.’s of three independent experiments (*P<0.05, **P<0.01; Student’st-test). Co-localization indexes were quantified for each ciliary cargo by counting at least 100 cilia. (g) Working model of MST1/2-SAV1 in ciliogenesis. See discussion for details. Figure 8: Depletion of MST1/2 and SAV1 impairs ciliary localization of ciliary proteins. ( a – d ) RPE cells were transduced with GFP-Rab8a ( a ), Smo-GFP ( b ) or GFP-RPGR ( c ). Each cell type was transfected with siRNA against MST1/2 or SAV1, and ciliogenesis was induced. Cells were co-immunostained for GFP ( a – c ) or Arl13b ( d ) and acetylated α- and γ-tubulin. γ-tubulin staining is presented only in merged images. Scale bar, 10 μm. ( e , f ) Ciliary localization indexes for Rab8a and RPGR were measured in AURKA and MST1/2-SAV1 co-depleted backgrounds. Error bars indicate s.e.m.’s of three independent experiments (* P <0.05, ** P <0.01; Student’s t -test). Co-localization indexes were quantified for each ciliary cargo by counting at least 100 cilia. ( g ) Working model of MST1/2-SAV1 in ciliogenesis. See discussion for details. Full size image In this study, we showed that the MST1/2–SAV1 complex, a component of the Hippo pathway, regulates ciliogenesis. MST1/2 was activated during ciliogenesis as indicated by increased phosphorylation of MST1 as well as MOB1, an established target of MST1 (ref. 18 ). Activated MST1/2 and SAV1 localized to the basal body of cilia and their loss impaired ciliogenesis in cell lines and a zebrafish model. The MST1/2–SAV1 complex promotes ciliogenesis by at least two independent mechanisms: inhibiting formation of the AURKA/HDAC6 cilia-disassembly complex and promoting ciliary localization of ciliary cargoes as a component of the NPHP transition-zone complex ( Fig. 8g ). AURKA activity during cilia disassembly is regulated by interactions with activating scaffold proteins, such as NEDD9, calmodulin or PIFO. Our results suggest that regulated interaction between AURKA and HDAC6 is another mechanism for controlling cilia disassembly. However, we still leave open the possibility that AURKA phosphorylation by MST1/2 also affects the interaction of AURKA with other regulatory proteins. We speculate that the target phosphorylation sites of AURKA by MST1/2 are multiple sites. The target phosphorylation sites in AURKA and how these phosphorylations affect the interaction of AURKA with HDAC6 remain to be determined in the future study. The NPHP and Tectonic complexes are responsible for the gating function of the transition zone as a membrane diffusion barrier [35] , [36] , [42] , [43] . Although proteomic studies have identified a massive number of components of the respective complexes, most of the identified components are scaffolding proteins without catalytic activities. The MST1/2–SAV1 complex might be one such enzyme that supports membrane diffusion barrier function of the transition zone as part of the NPHP complex. The substrate(s) of MST1/2 within the NPHP complex remain to be determined. MST1/2 might directly phosphorylate NPHP proteins, which in turn could serve as docking sites for other proteins. Another possibility is that NPHP proteins function as a large platform that recruits multiple proteins, including substrates of MST1/2. Several studies have suggested possible regulation of the Hippo pathway activity by NPHP proteins [40] , [44] , [45] . However, these experiments were conducted in nonciliated cells and did not investigate functional implication on ciliogenesis. Since some populations of NPHP proteins are observed at cell–cell junctions [30] , where the Hippo pathway is believed to be activated, we cannot completely rule out the possibility that the NPHP complex does affect YAP/TAZ activity in ciliated cells. However, based on our observation that SAV1 and NPHP1 co-localized at cilia and depletion of MST1/2–SAV1 decreased localization of established ciliary marker proteins to the axoneme, we would like to propose that the MST1/2–SAV1–NPHP complex contributes to the transition-zone function. While we have established the biological function of the MST1/2–SAV1–NPHP interaction, detailed biochemical interaction within the complex should be further characterized. Our results clearly demonstrate that SAV1 directly binds NPHP1 and MST1 interacts with NPHP1/4 indirectly via SAV1. Multiple lines of evidence support this conclusion. First, overexpression of SAV1 increased MST1–NPHP1/4 complex formation. Second, depletion of SAV1 reduced MST1–NPHP1/4 complex formation. Third, SAV1 directly bound NPHP1 but not NPHP4 in vitro , whereas MST1 bound none. We note that depletion of SAV1 or NPHP1 does not fully abolish MST1–NPHP1/4 or SAV1–NPHP4 complex, respectively. Incomplete knockdown likely explains this, although we cannot completely rule out the possibility that there are other scaffold proteins involved. Since NPHP1/4/8 proteins have many other interacting proteins, it is likely that multiple protein–protein interaction interfaces exist. Although complicated protein–protein interactions would constitute the full protein complex, MST1–SAV1–NPHP1 binding is clearly a part of the complex. One question arising from our data is the extent to which the two independent pathways mediated by MST1/2–SAV1 contribute to ciliogenesis. In cultured cells, depletion of AURKA perfectly rescued ciliogenesis, although the NPHP pathway is still affected. The most likely explanation is that the degree of impaired transition-zone function is below the threshold to actually reduce ciliogenesis. Our data show that the MST1/2–SAV1 complex is incorporated into the NPHP complex through interactions with NPHP1. While mutations of NPHP8 are found in patients with the most severe forms of ciliopathy, such as the Jourbert syndrome [46] , mutations in NPHP1 are mostly found in milder syndromes. In addition, depletion of NPHP1 in cultured cells or cells isolated from patients do not show impaired ciliogenesis [30] , [47] . In agreement with these reports, NPHP1 depletion did not impair ciliogenesis in our experimental system (data not shown). Notably, the sav1 morphant phenotype resembled that of the published Nphp1 morphant phenotype, with cardiac oedema and body-axis curving [30] . The extent to which the accelerated cilia disassembly through AURKA/HDAC6 in the absence of MST1/2–SAV1 contributes to ciliogenesis in vivo is not clear. We speculate that, since AURKA activity is tied up with multiple regulations, inhibition of cilia disassembly could be achieved by other compensatory mechanisms in vivo . Therefore, a secondary mutation might be required to unleash on-going cilia disassembly in vivo . The regulation of ciliogenesis by such cooperative interactions has been reported for VHL and GSK-3 (ref. 48 ). Moreover, the in vivo consequence of constitutive cilia disassembly itself is yet to be determined. Further genetic analyses are necessary to dissect the contribution of two pathways to ciliogenesis by MST1/2–SAV1 in vivo . It will be also important to examine whether Mst1/2 or Sav1 mutant mice show ciliopathy phenotypes. However, Mst1 or Mst2 single knockout mice are largely normal and double knockout mice are early embryonic lethal [27] , [28] , [49] . Sav1 conventional knockout mice also die before birth [50] . Therefore, the use of conditional knockout mice is necessary to assess ciliopathy phenotypes in these mutants. Notably, we observed that ~25% of Mst2 null mice in BL6/129 mixed background developed lethal hydrocephalus. Scanning electron microscope analysis of the brain showed scarce and shorter motile cilia in the affected mice (T.H. Kim and D.S. Lim, unpublished observations). This suggests that Mst1/2 (potentially Sav1) plays a role in ciliogenesis at least in this organ of mice. In summary, we found a role of MST1/2–SAV1 in inhibiting cilia disassembly and maintenance of cilia stability. We also propose a role of this complex in regulating localization of several ciliary proteins as component of the NPHP complex. What remains to be understood is whether the complex has a role in cilia assembly (early phase of ciliogenesis). To this end, we tested two early events of ciliogenesis in the absence of MST1/2–SAV1. Since these proteins are implicated in cell polarity, we examined whether centrosomes migrate normally in knockdown cells. Time course immunostaining with z-stack confocal imaging showed that centrosomes normally migrated upwards upon serum starvation in RPE cells ( Supplementary Fig. 14 ). We also investigated the localization of CP110. Presence of CP110 in centrioles blocks ciliogenesis and CP110 should disappear from the mother centriole to initiate ciliogenesis [51] . CP110 disappeared in the MST1/2–SAV1-depleted cells with comparable kinetics to control cells ( Supplementary Fig. 15 ). Although these two events were unaffected by MST1/2–SAV1 depletion, cilia assembly is a complicated process and it would be important to examine whether and how MST1/2–SAV1 contributes to this. In addition to our current findings, one recent study has proposed that NDR2 regulates trafficking of Rabin8, a guanine exchange factor for Rab8a (ref. 52 ). Since MST1/2 kinases are upstream activators of NDR1/2 kinases, it is also likely that MST1/2 contributes to ciliogenesis, in part, through NDR2. The emerging idea is that the MST1/2–NDR1/2 signalling system has an impact on microtubule-based cellular processes, whereas MST1/2–LATS1/2 signalling system regulates cell proliferation through the canonical Hippo pathway. It is well established that epithelial cell polarity regulates the Hippo pathway. However, whether the components of the Hippo pathway can regulate cell polarity processes apart from their role in controlling cell proliferation has not been investigated. Our current study shows that the Hippo pathway also controls cell polarity processes such as ciliogenesis. It has also been shown that Sav1-null villous enterocytes exhibit a loss of apical–basal polarity [50] . Since quiescent cells must disassemble their cilia for next mitosis, primary cilia can be considered tumour-suppressive organelles. Indeed, primary cilia are lost in aggressive human cancers [53] , [54] , and ciliogenesis has been shown to regulate tumorigenesis in mouse models [55] . Thus, our study provides another mechanism by which MST1/2 and SAV1 function as tumour suppressors. Another interesting topic for future investigation is whether and how primary cilia regulate Hippo pathway activity. YAP is inactivated by serum starvation and activated by Sphingosine-1-phosphate or lysophosphatidic acid components in serum [56] . Interestingly, Sphingosine-1-phosphate or lysophosphatidic acid signals via G protein-coupled receptors, many of which are known to localize to primary cilia. Therefore, it will be important to determine whether YAP regulation by serum depends on primary cilia and how it is altered in human cancers. Cell culture 293T cells were cultured in Dulbecco’s modified Eagle medium (DMEM) supplemented with 10% fetal bovine serum and penicillin/streptomycin. RPE and mIMCD3 cells were cultured in DMEM/F12 supplemented with 10% fetal bovine serum and penicillin/streptomycin. Stable RPE clones expressing HA-MST1 were established by transfecting RPE cells with pcDNA3 HA-MST1 followed by selection with 400 μg ml −1 of G418 for 2 weeks. All cell lines were purchased from ATCC and tested for mycoplasma contamination and validated as negative. Immunofluorescence Cytosolic acetylated α-tubulin background staining was minimized by first placing cells on ice for 45 min. Cells were then washed once with ice-cold PBS and fixed with ice-cold methanol. Blocking was carried out by incubating with 1% bovine serum albumin in PBS for 30 min at 4 °C. Primary antibodies were diluted in blocking buffer and incubated at 4 °C overnight. After washing three times with PBS, cells were incubated at 37 °C for 1 h with Alexa-488-, Alexa-594- or Cy5-conjugated secondary antibodies (diluted in PBS). Cells were then washed three times with PBS and mounted with mounting medium containing 4′,6-diamidino-2-phenylindole. While staining cilia for Arl13b, cells were directly fixed with ice-cold methanol without incubating on ice. For wheat germ agglutinin (WGA) labelling, live cells were labelled with Alexa-594-WGA as described by the manufacturer (Invitrogen). Cells were fixed with ice-cold methanol and proceeded as described above. Plasmids Rab8a and HDAC6 cDNAs were obtained from Addgene. NPHP4 and NPHP8 cDNAs were purchased from Kazusa DNA Research Institute and subcloned into pcDNA3.1 plasmids. NPHP1 and RPGR cDNAs were amplified from a human kidney cDNA library using the following primer pairs: NPHP1, 5′-GCGGATCCATGCTGGCGAGACGACAGCGA-3′ and 5′-GCCTCGAGTCACACTGCATTCTTTCTCATTTC-3′; RPGR, 5′-GCGGATCCATGAGGGAGCCGGAAGAGCTG-3′ and 5′-GCCTCGAGTTATAGTATTGTACAGGATTTTGAT-3′. siRNA and shRNA siRNA oligonucleotides were synthesized by Samchully Pharm. siRNA transfection was performed using Lipofectamine RNAiMAX (Invitrogen), as described by the manufacturer. shRNAs for lentiviral transduction were cloned into pLKO.1-puro or -hygro plasmids. Target sequences for siRNAs and shRNAs used in this study are available in Supplementary Table 1 . mRNA isolation and RT–PCR RNAs were isolated using Ribo-EX reagent (GeneAll), as described by the manufacturer. RNA samples (2 μg) were reverse-transcribed using 18(dT) oligo followed by manual PCR to detect target transcripts. The sequences of RT–PCR oligos used in this study were as follows: GAPDH forward, 5′-CTTCGCTCTCTGCTCCTCCT-3′; GAPDH reverse, 5′-GTTAAAAGCAGCCCTGGTGA-3′; TAO3 no. 1 forward, 5′-TGGGAAGCAGACCCATGAGAA-3′; TAO3 no. 1 reverse, 5′-TAATGGCAGCGATCTCCACTT-3′; TAO3 no. 2 forward, 5′-AACAGAGCCAGGTCAGGTAAA-3′; and TAO3 no. 2 reverse, 5′-TTCCGTTCCGCCAATTCAATA-3′. 3D acinar culture Chamber slides were coated with 0.235% NaHCO 3 and 3 mg ml −1 type I collagen in DMEM/F12. The collagen solution was solidified by incubating at 37 °C for at least 1 h without CO 2 . mIMCD3 cells (10 4 cells per slide) were resuspended in DMEM/F12 media containing 2% Matrigel and added on top of the collagen layer. Acini were allowed to develop for 4 days, and then were immunostained and analysed by Z-stack using confocal microscopy. Western blotting For western blot analysis, cells were lysed with lysis buffer containing 0.5% Triton X-100 or 1% NP-40, 50 mM Tris–Cl (pH 7.5), 150 mM NaCl, 1 mM EDTA and 1 mM MgCl 2 . Lysates were cleared by centrifugation for 30 min at 16,100 g , and protein concentration was measured using the Bradford assay. Lysates were fractionated by sodium dodecyl sulfate-polyacrylamide gel electrophoresis (SDS–PAGE) and transferred to nitrocellulose membranes. Membranes were blocked in 5% non-fat milk for 1 h and incubated with primary antibodies diluted in 5% non-fat milk or bovine serum albumin. Horseradish peroxide-linked secondary antibodies (Jackson Laboratory) were used at a 1:10,000 dilution (in milk), and blots were developed using an enhanced chemiluminescence (ECL) kit (Amersham). Full scans of all western blots and gels are supplied in Supplementary Fig. 16 . In vitro binding assay For in vitro binding assay, recombinant proteins or in vitro -translated proteins were mixed in TBS buffer (50 mM Tris–Cl, 150 mM NaCl) containing 0.1% Tween-20 and incubated overnight at 4 °C. Pull down was performed either by immunoprecipitation or using nickel beads (Qiagen) followed by three washes with binding buffer. GST-SAV1 and GST-AURKA proteins were purified from the Rosetta strain using GST affinity beads (Sigma). GST-MST1 and His-AURKA proteins were purchased from Abcam. In vitro -translation using the T7 promoter was performed as described by the manufacturer (Promega). Microinjection of mRNA and morpholino oligonucleotides Synthetic capped mRNAs of sav1 and sav1-EGFP were transcribed in vitro using the SP6 mMESSAGE mMACHINE Kit (Ambion). The synthesized mRNAs were dissolved in 0.2% Phenol Red, used as a tracking dye, and then microinjected into one- to two-cell stage embryos at 50 pg per embryo. For antisense knockdown experiments, sav1- ATG-MO (5′-CTGGAGAGCATTGTTAATCCGAATC-3), targeting the 5′-untranslated region, was synthesized by Gene Tools. Morpholinos were resuspended in 1 × Danieau’s buffer (58 mM NaCl, 0.7 mM KCl, 0.4 mM MgSO 4 , 0.6 mM Ca(NO 3 ) 2 , 5.0 mM HEPES, pH 7.6) containing 0.1% phenol red and then microinjected into one- to four-cell stage embryos (Danio rerio, WT) at 6 ng per embryo. No statistical method was used to predetermine sample size. All experiments were performed three times independently. Each embryo was randomly assigned to treatment groups. The investigators were not blinded to allocation during experiments and outcome assessment. All animal experiments were approved by the Animal Ethics Committee of Chungnam National University (CNU 00191). Whole-mount immunostaining of zebrafish For whole-mount immunostaining, zebrafish embryos were fixed in 4% paraformaldehyde. After three times washing with PBS supplemented with 0.1% Tween-20 (PBST), embryos were dehydrated with methanol, rehydrated and washed with PBST. Embryos were permeabilized in cold acetone for 8 min and washed with PBST. Blocking was carried out by incubating with 2% horse serum in PBST for 30 min at room temperature. Anti-acetylated α-tubulin antibody (Sigma, T7451; 1:1,000) were diluted in blocking solution and incubated at 4 °C overnight. After washing with PBST, embryos were incubated at 4 °C for 4 h with Alexa-568-conjugated secondary antibody (Invitrogen, A-11004; 1:500). Embryos were washed with PBST and mounted in 75% glycerol/PBST. Antibodies Antibodies against the following proteins were used in western blot analyses: MST1 (Cell Signaling, no. 3682), MST2 (Cell Signaling, no. 3952), phospho-MST1 (T183; Cell Signaling, no. 3681), phospho-pRB (S780; Cell Signaling, no. 9307), phospho-Cdc2 (Y15; Cell Signaling, no. 9111), YAP (Cell Signaling, no. 4912), phospho-YAP (S127; Cell Signaling, no. 4911), LATS2 (Cell Signaling, no. 5888), MOB1 (Cell Signaling, no. 3863), phospho-MOB1 (T35; Cell Signaling, no. 8699), LATS1 (Bethyl, A300–477A, 1:2,500), β-actin (Sigma, A5316, 1:10,000), cyclin A (Santa Cruz, sc-751), Myc (Santa Cruz, sc-40), GST (Santa Cruz, sc-138, 1:2,000), p27 (BD Biosciences, 554069), HA (Covance, MMS-101P, 1:2,500), HDAC6 (Millipore, 07–732 and Santa Cruz, sc-11420, 1:5,000) and Flag (WAKO, 012-22384). Rabbit anti-SAV1 (ref. 50 ; 1:2,500) and guinea pig anti-AURKA [57] (1:500) antibodies were previously described. Sheep anti-Tao1 antibody was a kind gift of Stephen Taylor. All antibodies of which dilution factors are not indicated were used in 1:1,000. Anti-AURKA antibody (BD Biosciences, 610938) and anti-MST1 antibody (Cell Signaling, no. 3682) were used for endogenous immunoprecipitation. Antibodies against the following proteins were used for immunofluorescence studies: acetylated α-tubulin (Sigma, T7451, 1:1,000), γ-tubulin (Sigma, T5192, 1:1,000), HA (Roche, 11867423001, 1:100), E-cadherin (BD Biosciences, 610182, 1:200), Ki67 (Novocastra, NCL-Ki67p, 1:200), CP110 (Proteintech, 12780-1-AP, 1:500) and Flag (WAKO, 012-22384, 1:200). The phospho-MST1 (T183) antibody (1:50) was generated by immunizing rabbits with CTMAKRNpTVIGTPF peptides. Guinea pig or rabbit anti-GFP serum (1:500) and rabbit anti-Arl13b serum (1:2,000) were kind gifts from Eunjoon Kim and Hyuk Wan Ko, respectively. BrdU- and EdU-incorporation assays EdU (10 μM) was added to cell media 30 min before fixation. EdU-incorporating cells were visualized using an EdU Alexa Fluor 594 Imaging Kit (Invitrogen), as directed by the manufacturer. BrdU (10 μM) was added to cell media 1 h before fixation. BrdU-incorporating cells were detected by monitoring the immunofluorescence of an anti-BrdU antibody (BD Biosciences). For this, cells were fixed with 4% paraformaldehyde (diluted in PBS) for 15 min followed by permeabilization with 0.2% Triton X-100 in PBS. Nuclei were disrupted by incubating with 2 N HCl for 15 min at 37 °C. Cells were neutralized with 0.1 M borate buffer (pH 8.5), followed by application of a conventional immunofluorescence procedure. Image acquisition and processing Images were collected with a ZEISS LSM 510 microscope using ZEISS C-Apochromat × 40/1.2 W and C-Apochromat × 63/1.2 W objectives and the ZEISS LSM 510 NLO acquisition software. For imaging ciliated cells, we always imaged roughly the same spots of coverslips in each experiment. The ImageJ software was used for subsequent image processing. For quantifying ciliogenesis indexes, only cells with acetylated α-tubulin emanating from γ-tubulin were regarded as positive. For quantification of ciliated cell frequency and cilia length, at least three independent experiments were performed with duplicate samples for each experiment. Statistical analysis Graphs were drawn using the GraphPad Prism software. For cilia length, we used the GraphPad Prism programme to test whether the distribution is Gaussian. We performed F-test (GraphPad Prism) to confirm that the variance is similar between the groups that are being statistically compared. Statistical analyses were done using paired two-tailed Student’s t -test with a 95% confidence interval. How to cite this article: Kim, M. et al. The MST1/2-SAV1 complex of the Hippo pathway promotes ciliogenesis. Nat. Commun. 5:5370 doi: 10.1038/ncomms6370 (2014).